On-demand optogenetic control of spontaneous seizures in temporal lobe epilepsy Temporal lobe epilepsy is the most common type of epilepsy in adults, is often medically refractory, and due to broad actions and long-time scales, current systemic treatments have major negative side-effects. However, temporal lobe seizures tend to arise from discrete regions before overt clinical behaviour, making temporally and spatially specific treatment theoretically possible. Here we report the arrest of spontaneous seizures using a real-time, closed-loop, response system and in vivo optogenetics in a mouse model of temporal lobe epilepsy. Either optogenetic inhibition of excitatory principal cells, or activation of a subpopulation of GABAergic cells representing <5% of hippocampal neurons, stops seizures rapidly upon light application. These results demonstrate that spontaneous temporal lobe seizures can be detected and terminated by modulating specific cell populations in a spatially restricted manner. A clinical approach built on these principles may overcome many of the side-effects of currently available treatment options. Epilepsy, a disorder of recurrent, spontaneous seizures actually comprises a number of distinct clinical disease entities, each with different phenotypes, underlying mechanisms, involved brain structures and prognoses [1] . In part because of their unpredictable nature, seizures can dramatically interfere with the daily lives of patients. This same feature poses an obvious challenge to the development of ideal therapeutic strategies that act only on an ‘as-needed’ basis, which would avoid disrupting normal interictal behaviours and reduce the frequently debilitating negative side-effects of currently available medications. Epilepsies are often categorized as being either generalized or partial. In generalized epilepsies such as absence epilepsy, seizures begin with an immediate change in level of consciousness, and electroencephalography (EEG) abnormalities appear across widespread brain areas simultaneously. In partial epilepsies such as temporal lobe epilepsy (TLE), however, early seizure activity appears in a restricted region and may or may not progress to involve the entire brain or affect level of consciousness [2] . This feature of TLE is clinically significant because it provides a theoretical time window for intervention between electrographic seizure onset and the onset of altered mental status. Thus, it is hypothetically possible to implement a temporally restricted therapeutic strategy for TLE and other partial epilepsies during early ictal activity, which could prevent consciousness-altering seizure progression without disrupting brain function during interictal time periods. While there is currently no Food and Drug Administration-approved on-demand treatment for epilepsy, clinical trials using closed-loop electrical stimulation have shown promise [3] . Optogenetic techniques provide immediate, temporary control of specific cell populations using light-sensitive opsins [4] , [5] , [6] , making them ideal candidates for on-demand seizure control. Indeed, in vitro and in vivo studies support the use of optogenetics to control seizure activity [7] , [8] , [9] . However, temporal specificity in epilepsy treatment additionally requires an accurate, fast method of detecting and responding to unpredictable seizures. This poses an additional challenge for on-demand treatment for TLE, because unlike in thalamocortical epilepsy, the electrographic appearance of seizures varies considerably between individuals. Additionally, the presence of interictal spiking makes rapid and selective detection of ictal events more challenging. We developed a novel, tunable closed-loop seizure-detection programme to identify and rapidly respond to seizures. Seizures were detected in real-time, triggering light delivery which was randomized, such that 50% of events received light and 50% served as no-light internal controls. When inhibitory opsins were expressed in excitatory principal cells, light application rapidly stopped seizures. Moreover, seizure control was also achieved when excitatory opsins were selectively expressed only in a subpopulation of inhibitory cells, which make up <5% of neurons in the hippocampus [10] , [11] . These results demonstrate that spontaneous temporal lobe seizures can be detected and stopped even by directly affecting only specific cell populations in a spatially restricted manner. The insight obtained from exploring seizure cessation by on-demand optogenetics provides an approach, based on direct modulation of a minimum number of cells and only at the time of a seizure, for the development of less disruptive interventions than are currently available for treating TLE. Real-time detection of spontaneous temporal lobe seizures To induce TLE in mice, we injected kainate (KA) unilaterally into the dorsal hippocampus. This model reproduces key features of unilateral human hippocampal sclerosis, ( Supplementary Fig. S1 ), and results in seizures that typically arise near the sclerotic region [12] , [13] , [14] . Both electrographic-only (little or no behavioural manifestations), as well as overtly behavioural (defined as minimally stage 3–4 on a modified Racine scale, with forelimb clonus plus rearing [15] ), spontaneous, recurrent seizures emerged over a period of weeks. We then implanted intrahippocampal depth electrodes and individual optical fibres (Methods). Seizures were detected using custom software ( Fig. 1 , detailed in Supplementary Methods and Supplementary Fig. S2 ). Briefly, detection was tuned to the specific EEG signature of the seizures in each chronically epileptic animal, using combinations of the following features: (1) signal power properties (magnitude, rate of change), (2) spike features (amplitude, width, rate, regularity) and (3) frequency properties (changes in energy within specific frequency bands). The tuning of the detection algorithm to each animal allowed us to quickly and accurately detect varying electrographic seizure morphologies and to intervene in real-time with both sensitivity and specificity ( Supplementary Note 1 ). 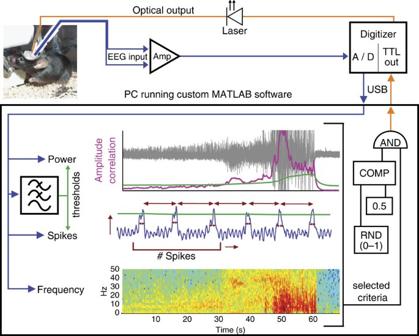Figure 1: Closed-loop system design. EEG input (blue) from the mouse hippocampus is amplified (Amp), digitized (A/D) and relayed to a PC running a custom-designed real-time seizure detection software. The signal is fed into a number of possible detection algorithms, which utilize features of signal power, spikes or frequency (sample schematics are presented here; detailed methodology is provided inSupplementary Methods). Thresholds for power and spike properties (green) are determined using tunable leaky integrators acting as low-pass filters. Top: Amplitude Correlation (purple, during an example seizure, shown in grey); Middle: spike characteristics (for example, amplitude, rate, regularity and spike width, shown in red); Bottom: power of the signal in specific frequency bands during the same seizure, with warmer colours representing higher energy. Once a seizure has been detected using the selected criteria, for 50% of the events in a random fashion (RND), the software activates the optical output (orange) delivered to the hippocampus of the mouse, via a TTL signal from the digitizer to the laser. All trigger events, however, are flagged for later off-line analysis. COMP, digital comparator. USB, universal serial bus. Figure 1: Closed-loop system design. EEG input (blue) from the mouse hippocampus is amplified (Amp), digitized (A/D) and relayed to a PC running a custom-designed real-time seizure detection software. The signal is fed into a number of possible detection algorithms, which utilize features of signal power, spikes or frequency (sample schematics are presented here; detailed methodology is provided in Supplementary Methods ). Thresholds for power and spike properties (green) are determined using tunable leaky integrators acting as low-pass filters. Top: Amplitude Correlation (purple, during an example seizure, shown in grey); Middle: spike characteristics (for example, amplitude, rate, regularity and spike width, shown in red); Bottom: power of the signal in specific frequency bands during the same seizure, with warmer colours representing higher energy. Once a seizure has been detected using the selected criteria, for 50% of the events in a random fashion (RND), the software activates the optical output (orange) delivered to the hippocampus of the mouse, via a TTL signal from the digitizer to the laser. All trigger events, however, are flagged for later off-line analysis. COMP, digital comparator. USB, universal serial bus. Full size image Direct inhibition of principal cells with halorhodopsin For opsin expression, we utilized two cell-type specific strategies expected to decrease principal cell activity. The first approach was to directly inhibit excitatory principal cells. We crossed mice expressing Cre under the calcium/calmodulin-dependent protein kinase II alpha promoter (CamK-Cre [16] ) with mice expressing the inhibitory opsin halorhodopsin (HR) Cre-dependently (Ai39 (ref. 17 )) to generate animals-expressing HR in CamKII-expressing cells (Cam-HR mice). We utilized a single optical fibre placed just dorsal to the ipsilateral hippocampus near the site of KA injection to deliver light (amber, 589 nm) to a limited volume of tissue (estimated volume: <0.1 mm 3 , Methods). This effectively controlled electrographic seizures in all Cam-HR animals tested ( n =6 animals, P <0.01 for each animal, two-sample Kolmogorov–Smirnov (K–S) and two-tailed Mann–Whitney (M–W) tests, Fig. 2 ). On average, 57±12% of seizures stopped within 1 s of light delivery, and seizure duration postdetection was reduced by 70±8% (‘duration reduction’; seizure duration light versus no-light, n =6 animals: P <0.05, Wilcoxon test; duration reduction in opsin expressing, n =6 animals, versus negative controls, n =3 animals: P <0.05, M–W; Fig. 2g–i ). This indicates that temporal lobe seizures can be stopped by appropriately timed and, importantly, spatially restricted intervention. 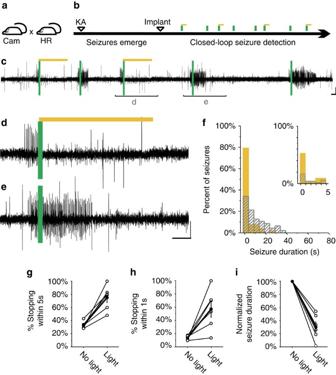Figure 2: Seizure control in mice-expressing HR in principal cells in a model of TLE. (a) Crossing CamK-Cre and Cre-dependent HR mouse lines generated mice expressing the inhibitory opsin HR in excitatory cells (Cam-HR mice). (b) Experimental timeline. (c–e) Example electrographic seizures detected (vertical green bars), activating amber light (589 nm) randomly for 50% of events (light: amber line, example ind; no-light example ine). (f) Typical example distribution of postdetection seizure durations (5 s bin size) during light (solid amber) and no-light internal control conditions (hashed grey). Inset: first 5 s bin expanded, 1 s bin size. Note that most seizures stop within 1 s of light delivery. (g–i) Group Cam-HR data showing the per cent of seizures stopping within 5 s of detection (g), within 1 s of detection (h), and the average postdetection seizure duration (normalized to average no-light postdetection duration for each animal) (i). Note that in one animal (shown inc–e), all seizures were stopped within 1 s of light delivery. Averaged data: filled circles. Error bars represent s.e.m. Scale bars inc–e, 100 μV, 5 s. Figure 2: Seizure control in mice-expressing HR in principal cells in a model of TLE. ( a ) Crossing CamK-Cre and Cre-dependent HR mouse lines generated mice expressing the inhibitory opsin HR in excitatory cells (Cam-HR mice). ( b ) Experimental timeline. ( c – e ) Example electrographic seizures detected (vertical green bars), activating amber light (589 nm) randomly for 50% of events (light: amber line, example in d ; no-light example in e ). ( f ) Typical example distribution of postdetection seizure durations (5 s bin size) during light (solid amber) and no-light internal control conditions (hashed grey). Inset: first 5 s bin expanded, 1 s bin size. Note that most seizures stop within 1 s of light delivery. ( g – i ) Group Cam-HR data showing the per cent of seizures stopping within 5 s of detection ( g ), within 1 s of detection ( h ), and the average postdetection seizure duration (normalized to average no-light postdetection duration for each animal) ( i ). Note that in one animal (shown in c – e ), all seizures were stopped within 1 s of light delivery. Averaged data: filled circles. Error bars represent s.e.m. Scale bars in c – e , 100 μV, 5 s. Full size image Although off-peak for the activation spectrum of HR, red light, which has greater tissue penetration, has been shown in vitro to activate HR [6] , [17] . In Cam-HR animals in vivo , red light (635 nm) significantly controlled seizures, with a 57±14% duration reduction, and 46±12% stopping within 1 s (significant duration reduction in 3 of 3 animals, P <0.01 each, K–S and M-W). This indicates the clinical potential for using red light with future optogenetic therapies, which not only could reach a larger volume of tissue, but may also eventually allow light to be delivered less invasively (that is, especially with the continued advancement of red-shifted opsins [6] , [18] , it may be possible to reach even deep tissue transcranially). Finally, as a large per cent of seizures were stopped within 5 s of light delivery, we examined whether similar seizure control could also be obtained while delivering light over a shorter time frame. Not unexpectedly, the per cent of seizures stopping within 5 s was not affected by the reduction in light duration; there was also no significant impact on seizure duration reduction (per cent stopping within 5 s of light: 58±8% with 30 s of light; 58±12% with 10 s of light, P =1, Wilcoxon; duration reduction: 53±7% with 30 s of light; 42±12% with 10 s of light, P =0.6, Wilcoxon; n =4). Excitation of inhibitory PV-containing GABAergic cells The second cell-type specific strategy we tested for stopping seizures was to activate a subpopulation of GABAergic cells. Although parvalbumin (PV)-containing cells represent <5% of hippocampal neurons [10] , [11] , PV-containing cells are known to have a major role in synchronizing principal cell populations during gamma oscillations [19] , [20] , [21] , and individual PV-containing cells can contact over 1,000 pyramidal cells in CA1 ( [10] ). Therefore, we asked whether the coordinated activation of PV cells could exacerbate the synchronous discharge of neurons [20] during seizures and thus potentially prolong them, or alternatively, if their inhibition of principal cells could reduce seizure duration. Selective expression of excitatory channelrhodopsin (ChR2) in PV-containing GABAergic cells was achieved by crossing PV-Cre mice [22] with mice-expressing ChR2 Cre-dependently (Ai32 (ref. 17 )) ( Fig. 3 ). Light delivery (blue, 473 nm) to the hippocampus ipsilateral to KA injection in PV-ChR2 mice significantly shortened seizures: 43±11% duration reduction, 59±11% stopping within 5 s of light delivery (seizure duration light versus no-light, n =8 animals, P <0.05, M-W; at the individual animal level, 5 of 8 animals showed a significant effect, P <0.05 each, M-W and K–S tests, Fig. 3c ). This indicates that opsin-mediated activation of PV cells does not exacerbate, but instead curtails seizures. Moreover, these findings demonstrate that not only can a temporally and spatially restricted treatment approach control seizures, but also that a more cell-type specific approach, directly affecting only a small proportion of neurons within the area of illumination, can provide significant seizure control. 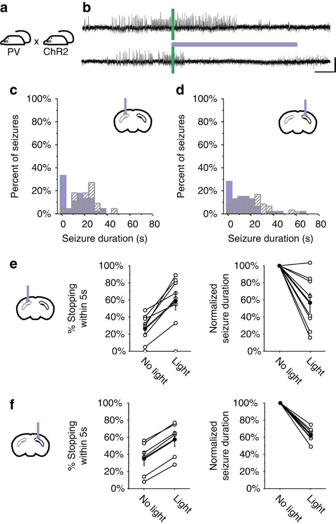Figure 3: Ipsilateral and contralateral control of seizures in PV-ChR2 mice. (a) Crossing PV-Cre and Cre-dependent ChR2 mouse lines generated mice expressing the excitatory opsin ChR2 in PV-expressing GABAergic cells (PV-ChR2 mice). (b) Example electrographic seizures in a PV-ChR2 mouse (top, no-light) truncated by blue (473 nm) light delivery (bottom, blue line) to the hippocampus. (c) Distributions of postdetection seizure durations from the same animal during light and no-light conditions (solid blue: light; hashed grey: no-light), when light was delivered (blue probe) ipsilateral to the KA injection (grey hemisphere). (d) In the same animal, light delivered instead to the hippocampus contralateral to KA injection also shortens electrographic seizures. (e–f) Group data for PV-ChR2 animals with light delivered ipsilateral (e) or contralateral (f) to the KA injection site. Electrographic recordings were consistently from the hippocampus ipsilateral to KA injection. Averaged data: filled circles. Error bars represent s.e.m. Figure 3: Ipsilateral and contralateral control of seizures in PV-ChR2 mice. ( a ) Crossing PV-Cre and Cre-dependent ChR2 mouse lines generated mice expressing the excitatory opsin ChR2 in PV-expressing GABAergic cells (PV-ChR2 mice). ( b ) Example electrographic seizures in a PV-ChR2 mouse (top, no-light) truncated by blue (473 nm) light delivery (bottom, blue line) to the hippocampus. ( c ) Distributions of postdetection seizure durations from the same animal during light and no-light conditions (solid blue: light; hashed grey: no-light), when light was delivered (blue probe) ipsilateral to the KA injection (grey hemisphere). ( d ) In the same animal, light delivered instead to the hippocampus contralateral to KA injection also shortens electrographic seizures. ( e – f ) Group data for PV-ChR2 animals with light delivered ipsilateral ( e ) or contralateral ( f ) to the KA injection site. Electrographic recordings were consistently from the hippocampus ipsilateral to KA injection. Averaged data: filled circles. Error bars represent s.e.m. Full size image Approximately 60% of seizures in the intrahippocampal KA model start in the hippocampus ipsilateral to KA injection [12] . In this model, as well as in human epileptic patients, a proportion of seizures can also arise from the contralateral hippocampus, sometimes referred to as a ‘mirror focus’ [12] , [23] . We, therefore, tested the effect of light delivery to the contralateral hippocampus of PV-ChR2 mice. Although the electrographic seizures were recorded in the hippocampus ipsilateral to KA injection, contralateral light still significantly suppressed seizures (37±4% duration reduction, 58±8% stopping within 5 s; seizure duration light versus no-light, n =6 animals: P <0.05, Wilcoxon; 5 of 6 animals showed a significant reduction at the individual animal level, K–S and M-W; Fig. 3d ). Indeed, opsin activation significantly reduced seizure duration in a comparable fashion when light was delivered to the hippocampus either ipsilateral or contralateral to KA injection and electrode placement (ipsilateral versus contralateral light stimulation P =0.51; opsin-expressing versus opsin-negative littermate controls P <0.05; two-way analysis of variance, Holm–Bonferroni test; n =11 opsin-negative littermate control animals, 10 tested ipsilateral, 9 tested contralateral to KA injection; no interaction, P =0.89). These results demonstrate that the ipsilateral hippocampus is not the only potential target for optogenetic intervention. Importantly, because seizures were detected from one hemisphere, and light delivered to the other, this further demonstrated that the effect of light on seizures was not confined to the region directly illuminated by the optical fibre, and suggests that contralateral connexions are important in ongoing seizure activity in vivo . Opsin-mediated cellular effects of light stimulation Successful seizure intervention with opsin expression limited to PV-expressing neurons prompted us to consider the likely extent of our on-demand intervention in vivo . Note that not only was opsin expression in these animals limited to a fraction of neurons (<5%), but also the light intervention was spatially restricted. Given the average power measured post hoc from the tips of implanted fibres (9.7±1.5 mW), and the reported irradiance values required for activating opsins [6] , [24] , we estimate that sufficient blue light reached a depth of <1 mm in these animals ( Fig. 4a ). Moreover, with the on-demand application of brief pulses of light that we used in our experiments, it does not appear that PV cells are driven to fire beyond physiological firing rates, as we did not observe an increase in the number or proportion of PV cells expressing c-Fos (an immediate early gene activated in response to increased cell activity) following 2 h of on-demand stimulation as used in our experiments (c-Fos expression was found in only 4 of 316 PV cells; Fig. 4b ). However, if we used an extreme paradigm of continuous light pulses (50 ms on, 100 ms off) for 2 h, rather than only on-demand at the time of seizures, we observed a marked increase in c-Fos expression in PV cells (286 of 475 PV cells). Note that this increase in c-Fos expression in PV cells was only seen in PV-ChR2 opsin-expressing, and not PV-ChR2 opsin-negative control animals also receiving such an extreme light paradigm (opsin-negative: 5 of 430 PV cells expressed c-Fos; Fig. 4b ). 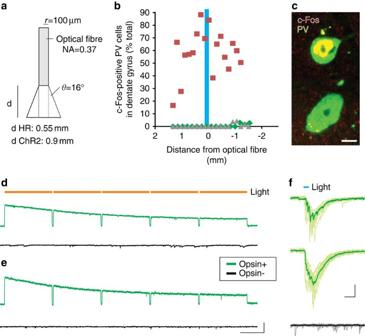Figure 4: Extent and specificity of light-activation of opsin-expressing cells. (a) Diagram of illumination. The fibres used in this study have a numerical aperture (NA) of 0.37 and a radius (r) of 100 μm. With an index of refraction (n) for brain tissue of 1.35, and a flat cleave tip, there is a half-angle (θ) of ~16°. Given our average power measuredpost hocfrom the implanted fibre tip, and reported irradiance values for activating opsins, we reach a depth (d) of 0.55 mm for HR with amber light and 0.9 mm for ChR2 with blue light. Note that the diagram is not drawn to scale. (b) c-Fos expression is not induced in PV cells after 2 h of on-demand light (green diamonds), but can be induced with continuously pulsed blue light for the entire 2 h (that is, not on-demand light application, red squares) in PV-ChR2 opsin-expressing animals. Note that this c-Fos expression induced by 2 h long pulsed light application reflects both direct and indirect activation over a prolonged time period (for example, through gap-junctions and network connexions). An increase in PV-cell c-Fos expression was not observed without opsin expression (grey triangles). Light was delivered, and c-Fos expression examined, contralateral to the site of KA injections. (c) Example PV cells from PV-ChR2 opsin-expressing (top) and opsin-negative (bottom) animals inb. Green: PV. Red: c-Fos. Yellow: co-localization. Scale bar, 10 μm. (d,e) Long pulses of light (2 s on, 50 ms off; orange bars) produced robust outward (inhibitory) currents in CA1 pyramidal (d) and granule cells (e) of epileptic Cam-HR opsin-expressing animals (green traces), but not epileptic opsin-negative littermate controls (black traces). Scale bars, 1 s, 100 pA. Holding potential, −60 mV. (f) A single pulse of light (10 ms) produces robust postsynaptic currents in two CA1 pyramidal cells (dual recording) from a KA-treated PV-ChR2 opsin-expressing animal (green bolded trace, average of 15 individual sweeps, shown in light green). No-light-induced responses were seen in opsin-negative animals (bottom, average trace shown in black). Scale bars, 20 ms, 40 pA. Holding potential, −80 mV. Figure 4: Extent and specificity of light-activation of opsin-expressing cells. ( a ) Diagram of illumination. The fibres used in this study have a numerical aperture (NA) of 0.37 and a radius ( r ) of 100 μm. With an index of refraction ( n ) for brain tissue of 1.35, and a flat cleave tip, there is a half-angle ( θ ) of ~16°. Given our average power measured post hoc from the implanted fibre tip, and reported irradiance values for activating opsins, we reach a depth (d) of 0.55 mm for HR with amber light and 0.9 mm for ChR2 with blue light. Note that the diagram is not drawn to scale. ( b ) c-Fos expression is not induced in PV cells after 2 h of on-demand light (green diamonds), but can be induced with continuously pulsed blue light for the entire 2 h (that is, not on-demand light application, red squares) in PV-ChR2 opsin-expressing animals. Note that this c-Fos expression induced by 2 h long pulsed light application reflects both direct and indirect activation over a prolonged time period (for example, through gap-junctions and network connexions). An increase in PV-cell c-Fos expression was not observed without opsin expression (grey triangles). Light was delivered, and c-Fos expression examined, contralateral to the site of KA injections. ( c ) Example PV cells from PV-ChR2 opsin-expressing (top) and opsin-negative (bottom) animals in b . Green: PV. Red: c-Fos. Yellow: co-localization. Scale bar, 10 μm. ( d , e ) Long pulses of light (2 s on, 50 ms off; orange bars) produced robust outward (inhibitory) currents in CA1 pyramidal ( d ) and granule cells ( e ) of epileptic Cam-HR opsin-expressing animals (green traces), but not epileptic opsin-negative littermate controls (black traces). Scale bars, 1 s, 100 pA. Holding potential, −60 mV. ( f ) A single pulse of light (10 ms) produces robust postsynaptic currents in two CA1 pyramidal cells (dual recording) from a KA-treated PV-ChR2 opsin-expressing animal (green bolded trace, average of 15 individual sweeps, shown in light green). No-light-induced responses were seen in opsin-negative animals (bottom, average trace shown in black). Scale bars, 20 ms, 40 pA. Holding potential, −80 mV. Full size image To further address the specificity of light-mediated currents, we performed whole-cell patch-clamp recordings from hippocampal slices prepared from opsin-expressing and opsin-negative epileptic animals of both genotypes. In Cam-HR animals, principal cells in opsin-expressing animals responded to light with sustained outward currents, while no currents were induced in cells of opsin-negative animals ( Fig. 4d ). Similarly, in principal cells of PV-ChR2 opsin-expressing animals, light pulses induced inhibitory postsynaptic currents due to the activation of presynaptic PV cells, while no currents were induced in neurons from opsin-negative animals ( Fig. 4f ). On-demand intervention reduces behavioural seizure frequency We next examined whether stopping electrographic seizures can affect progression to overt behavioural seizures. Overall, light produced a 29.6% reduction in behavioural seizures ( n =184 seizures from 9 animals, P <0.05, χ 2 ; an example animal is shown in Fig. 5 ). This reduction occurs despite the observation that in the intrahippocampal KA model of TLE 27% of seizures either start outside of the hippocampus or have diffuse areas of onset [12] ; these seizures may be especially resistant to focal intervention. Taken together, our results indicate that optogenetic techniques can provide on-demand seizure control for electrographic seizures and reduce the frequency of behavioural seizures. 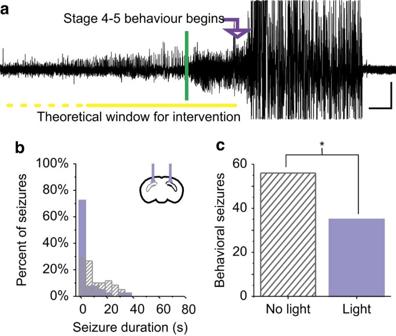Figure 5: Reduction in behavioural seizure frequency. (a) Example behavioural (stage 5) seizure (movement artifacts truncated). The vertical green bar indicates online seizure detection, prior to the start of stage 4–5 behaviour (arrow). The yellow bars under the trace highlight the theoretical window for intervention. Scale bars, 100 μV, 5 s. (b) Distribution of electrographic seizure duration after detection with (blue bars) and without (grey hashed bars) bilateral light intervention. Note that for behavioural seizure experiments in two animals light was delivered bilaterally. (c) Significant reduction in the frequency of behavioural seizures occurring during light compared with no-light (example animal; asterisk,P<0.05, two-tailed binomial). Electrographic recordings were consistently from the hippocampus ipsilateral to KA injection. Same mouse as shown in examples inFigure 3. Figure 5: Reduction in behavioural seizure frequency. ( a ) Example behavioural (stage 5) seizure (movement artifacts truncated). The vertical green bar indicates online seizure detection, prior to the start of stage 4–5 behaviour (arrow). The yellow bars under the trace highlight the theoretical window for intervention. Scale bars, 100 μV, 5 s. ( b ) Distribution of electrographic seizure duration after detection with (blue bars) and without (grey hashed bars) bilateral light intervention. Note that for behavioural seizure experiments in two animals light was delivered bilaterally. ( c ) Significant reduction in the frequency of behavioural seizures occurring during light compared with no-light (example animal; asterisk, P <0.05, two-tailed binomial). Electrographic recordings were consistently from the hippocampus ipsilateral to KA injection. Same mouse as shown in examples in Figure 3 . Full size image In this paper, we demonstrate that spontaneous temporal lobe seizures can be detected in real-time, and that spatially restricted intervention can stop seizures. This is shown using two distinct optogenetic approaches. First, using HR to directly inhibit principle cells, and second, using ChR2 to excite PV-expressing GABAergic neurons. In this latter approach, despite the fact that <5% of the illuminated neuronal population was directly affected by light intervention, significant seizure control was still achieved, stopping electrographic seizures and reducing the frequency of behavioural seizures. These results demonstrate a potential for using optogenetics with closed-loop seizure detection for a real-time, spatially restricted, therapeutic intervention to control spontaneous seizures in TLE. TLE is the most common type of epilepsy in adults. Recently, optogenetic techniques have been applied in models of other types of epilepsy, namely focal cortical epilepsy [8] and stroke-induced thalamocortical epilepsy [9] , supporting the general applicability of optogenetic approaches to stopping seizures, despite diverse underlying pathophysiologies. Importantly, we demonstrate not only that TLE is amenable to optogenetic intervention, but also that such intervention can be achieved when targeting opsins to specific, very restricted cell populations. Indeed, a major benefit of optogenetic approaches compared with currently available electrical stimulation devices is cell-type specificity. In this regard, optogenetic techniques can be considered not only as opportunities to develop treatment options directly, but also as a tool to better understand the basic mechanisms of seizures and to identify cell populations that might be more specifically targeted pharmacologically. Optogenetics thus provides a means to further our understanding of the roles of specific cell types in seizure generation and cessation. There is intense interest in developing a closed-loop, on-demand, system for the treatment of epilepsy, due to the potential outcome benefits of such temporally specific treatment. Online seizure detection is more challenging in TLE than in thalamocortical epilepsies; however, early intervention during seizures is especially clinically relevant for TLE, as detection is possible before generalization and altered levels of consciousness. Online seizure detection has been reported in rodent models of epilepsy [9] , [25] , [26] , as well as in clinical trials [3] . The combination of online seizure detection and optogenetic control of temporal lobe seizures described here may prove particularly powerful for future therapeutics, allowing for a spatially, temporally and cell-type selective intervention before overt clinical behaviour. Animals The molecular Cre-lox system permitted the expression of genetically introduced ChR2, or HR in specific cell populations. Mice were generated by crossing Cre lines-expressing Cre either in principal cells (CamK-Cre; B6.Cg-Tg(Camk2a-cre)T29-1Stl/J; stock 005359 from Jackson labs [16] ) or in PV-containing GABAergic interneurons, including bistratified cells, fast-spiking basket cells and axo-axonic (chandelier) cells [10] , [27] , [28] , [29] (PV-Cre;B6;129P2-Pvalbtm1(Cre)Arbr/J; stock 008069 from Jackson labs [22] ), with either floxed-STOP ChR mice (Ai32; Rosa-CAG-LSLChR2H134R-EYFP-deltaNeo generated by Hongkui Zeng, obtained from the Allen Institute; Ai32D is now available from Jackson labs, stock 012569 (ref. 17 )) or floxed-STOP HR mice (Ai39; B6;129S-Gt(ROSA)26Sortm39(CAGHOP/EYFP)Hze/J; generated by Hongkui Zeng, available from Jackson labs, stock 014539 (ref. 17 ), maintained by crossing with C57BL/6J mice). These crosses generated mice-expressing ChR in all PV-containing cells (PV-ChR) and mice-expressing HR in principal cells (Cam-HR). Ospin-negative littermates were used as non-expressing controls. Epilepsy induction and monitoring All procedures were approved by the UC Irvine Animal Care and Use Committee. Surgical procedures were performed stereotaxically under isofluorane anaesthesia and local nerve block induced by 0.5% bupivacaine. Kainic acid (50–100 nl, 20 mM in saline, Tocris Bioscience) was injected into the left dorsal hippocampus (2.0 mm posterior, 1.25 mm left, and 1.6 mm ventral to bregma) of mice on or after postnatal day 46. After recovery, animals were returned to the vivarium for at least 2 weeks to allow for the emergence of spontaneous recurrent seizures. Bipolar depth electrodes (PlasticsOne) and optical fibres (0.37NA, Low OH, 200 μm diameter, ThorLabs) terminated in 1.25 mm ceramic ferrules (Kientec Systems, Inc.) were implanted ipsilaterally (posterior 2.5 mm, left 1.75 mm, ventral 1.25 mm with respect to bregma) and in some cases, also contralaterally at the same posteroventral position into the hippocampus, targeting the dorsal stratum oriens of the CA1 such that emitted light would illuminate the hippocampal formation. Optical fibres and electrodes were fixed to the skull using screws (McMaster-Carr) and dental cement (Teets Cold Curing) and the animals were allowed to recover for several days before beginning 24-h video and EEG monitoring for seizures and subsequent closed-loop seizure detection and light delivery. On average, animals were implanted 15±2.3 weeks after KA injection and the effect of light on seizures was examined 15.9±1.4 weeks after KA injection (range: 2.4–24.6 weeks). There was no correlation between seizure duration reduction and time since KA for either Cam-HR or PV-ChR2 mice ( P =0.39 and P =0.83, respectively, Spearman test; see also Supplementary Fig. S3 ). Closed-loop seizure detection and light delivery Following the implant procedure, animals were connected through an electrical commutator (PlasticsOne) to an analogue Brownlee 410 amplifier; signals were digitized by an NI USB-6221-BNC digitizer (National Instruments) sampled at 500 Hz, and analysed in real-time by a PC running a custom MATLAB seizure detection algorithm (see below). Animals were also connected to a fibre-coupled diode laser (Shanghai Laser & Optics Century Co., Ltd) of an appropriate wavelength to activate the opsin expressed (blue=473 nm, amber=589 nm, or red=635 nm). Optical patch cords (Thorlabs, Doric Lenses) directed the laser light to the mouse through an optical commutator (Doric lenses), and were terminated in a 1.25 mm ferrule, which was connected to the implanted optical fibre with a ceramic split sleeve (Precision Fibre Products, Inc.). Average laser power at the source was 33±3 mW and the final power at the tips of the implanted optical fibres (measured post hoc ) was 9.7±1.5 mW. Continuous video and EEG monitoring established the presence of spontaneous recurrent seizures in individual animals, at which time an experimenter used custom MATLAB software to identify features of the early ictal electrographic signal to be used in triggering the real-time closed-loop seizure detection software. The experimenter could select from a number of different inclusion or exclusion criteria and could adjust thresholds to optimally detect the seizures with maximum sensitivity and specificity. Briefly, the following features could be used alone or in combination to tune the seizure detection algorithm (see Supplementary Methods for additional details): (1) signal power properties (magnitude, rate of change), (2) spike features (amplitude, width, rate, regularity) and (3) frequency properties (changes in energy within specific frequency bands). Note that a simple spike detection algorithm (for example, ref. 25 ) would be insufficient in this model of epilepsy. Once tuned, the custom closed-loop MATLAB software was used to activate the laser in real-time during seizures. When the specified criteria were met, the detector triggered, flagging the event for later review and in 50% of cases (in random sequence) immediately triggered the activation of the laser connected to the animal. Either short light pulses (50 ms on, 100 ms off) or long light pulses (2,000 ms on, 50 ms off) for 30–60 s, unless otherwise noted in the text, were used to activate the opsins. Histology For histological experiments, animals were deeply anaesthetized and perfused with paraformaldehyde (for c-Fos experiments, this occurred immediately following the 2 h stimulation period), coronal sections were made and either stained for c-Fos and PV (goat anti-parvalbumin PVG-214, Swant; rabbit anti-c-Fos (4): sc-52, Santa Cruz Biotechnology), or using a standard Nissl protocol. PV and c-Fos expression were examined from 50 μm sections every 200 μm throughout the entire anterior–posterior extent of the hippocampus. For entorhinal cortical histology, horizontal sections were made and stained using a fluorescent Nissl stain (Molecular Probes, N-21479) prepared as per the manufacturer’s instructions. Slice electrophysiology Whole-cell patch-clamp recordings were made from coronal slices ipsilateral to the site of KA injection at 36 °C in artificial cerebrospinal fluid containing (in mM) 2.5 KCl, 10 Glucose, 126 NaCl, 1.25 NaH 2 PO 4 , 2 MgCl 2 , 2 CaCl 2 , 26 NaHCO 3 ; with intracellular solution containing (in mM) 90 potassium gluconate, 27.4 KCl, 1.8 NaCl, 1.7 MgCl 2 , 0.05 EGTA, 10 HEPES, 2 Mg-ATP, 0.4 Na 2 -GTP, 10 phosphocreatine, 8 biocytin; pH 7.2; 270–290 mOsm; pipette resistance: 3–4.5 MΩ. Light was delivered through the epifluorscence port of a Nikon Eclipse FN-1, using a Lambda DG-4 with smart shutter and LAMDA SC controller (Shutter Instruments), and TTL input from a Digidata 1322A (Axon Instruments). Estimation of the tissue volume directly affected by light The fibres used in this study have a numerical aperture of 0.37, and a radius of 100 μm. With an index of refraction for brain tissue of 1.35 ( [30] ), and a flat cleave tip, there is a half-angle of ~16°. Given our average power measured post hoc from the implanted fibre tip (9.7 mW), and reported irradiance values capable of activating opsins (3.5 mW/mm 2 for HR [6] ; 1 mW/mm 2 for ChR2 ( [24] )), we reach a depth of 0.55 mm for HR with amber light and 0.9 mm for ChR2 with blue light (Deisseroth Lab online light transmission calculator, http://www.stanford.edu/group/dlab/cgi-bin/graph/chart.php ). With the simplification of even light at the end of the cone, this translates into a cone volume of 0.16 mm 3 for ChR2 and 0.06 mm 3 for HR. Statistical analysis Electrographic seizure duration before and after the time of the trigger was analysed off-line by reviewers blinded to the light condition and genotype of the animal, and behavioural seizures were confirmed by video and EEG analysis. Seizure duration distributions for light and no-light conditions were compared in each animal using a two-sample Kolmogorov–Smirnov test, and seizure durations were compared using a two-tailed Mann–Whitney test. Effects on seizure duration at the group level were tested using a Wilcoxon Signed Ranks Test. Comparison of reduction in seizure duration between conditions for PV-ChR2 animals (light location and opsin expression) was made using a two-way analysis of variance with Bonferroni-Holm tests. An effect of light on behavioural seizure frequency was evaluated with a two-tailed χ 2 -test. Only appropriately timed triggers for behavioural seizures (that is, triggers during the electrographic-only portion of the seizure, before, but within 60 s of the emergence of overt behaviour) were included in the final analysis. Values presented are mean±s.e.m. A P -value <0.05 was considered significant. Statistical analysis was done using Microsoft Excel 2007, OriginPro 8 and Google documents. How to cite this article: Krook-Magnuson, E. et al. On-demand optogenetic control of spontaneous seizures in temporal lobe epilepsy. Nat. Commun. 4:1376 doi: 10.1038/ncomms2376 (2013).